Electric-field control of magnetic domain-wall velocity in ultrathin cobalt with perpendicular magnetization Controlling the displacement of a magnetic domain wall is potentially useful for information processing in magnetic non-volatile memories and logic devices. A magnetic domain wall can be moved by applying an external magnetic field and/or electric current, and its velocity depends on their magnitudes. Here we show that the applying an electric field can change the velocity of a magnetic domain wall significantly. A field-effect device, consisting of a top-gate electrode, a dielectric insulator layer, and a wire-shaped ferromagnetic Co/Pt thin layer with perpendicular anisotropy, was used to observe it in a finite magnetic field. We found that the application of the electric fields in the range of ±2–3 MV cm −1 can change the magnetic domain wall velocity in its creep regime (10 6 –10 3 m s −1 ) by more than an order of magnitude. This significant change is due to electrical modulation of the energy barrier for the magnetic domain wall motion. Magnetic domain wall (DW) motion has been intensively investigated from the viewpoints of both physics and potential applications [1] , [2] , [3] , [4] , [5] , [6] , [7] , [8] , [9] , [10] , [11] , [12] , [13] , [14] , [15] , [16] , [17] , [18] , [19] , [20] , [21] . Current-induced DW motion is of particular interest because it enables the position of DW to be controlled electrically without applying an external magnetic field [1] , [2] , [3] , [4] , [7] , [8] , [9] , [10] , [11] , [12] , [13] , [14] , [16] , [17] , [18] , [19] , [20] , [21] . The electric field effect on magnetic materials has been actively studied recently, because magnetic properties can be controlled electrically [22] , [23] , [24] , [25] , [26] , [27] , [28] , [29] , [30] , [31] , [32] , [33] , [34] , [35] , [36] , [37] , when a field-effect-device structure—that is, one consisting of a top-gate electrode, a dielectric insulator layer (or a liquid electrolyte), and a ferromagnetic layer—is used to modulate a carrier density. The first reported magnetic phase transition induced by the electric field was one in a ferromagnetic semiconductor [22] . Electric-field control of coercivity [25] DW propagation [27] magnetic anisotropy [29] (magnetization direction), and magnetization [31] have also been reported. More recently, similar effects have been observed even in ferromagnetic metals at room temperature [30] , [32] , [33] , [34] , [36] , [37] , and these effects are attracting much attention owing to their potential use in practical applications. In this paper, we show the electric field effect, at room temperature, on the velocity of a single DW propagating in a micrometer-scale wire made of Co. The observed significant change in the velocity was found to be due to the electrical modulation of the effective energy barrier for the thermally activated DW creep motion [18] , [19] , [38] , [39] , [40] , [41] . Device structure and hall measurement A perpendicularly magnetized Co/Pt system [21] , [37] , [38] , [39] , [40] , [42] was used in the work reported here. The Co and the Pt layers were deposited on a semi-insulating GaAs substrate (see Methods for film deposition and layer structure). We made two sample devices with the same Co thickness (0.4 nm) but different Pt thicknesses (1.04 nm for sample 1 and 1.20 nm for sample 2). The field-effect device we fabricated, a 20-μm-wide Co wire with two Hall probes (A and B), is shown schematically in Fig. 1a (see Methods for the device fabrication). The gate voltage V G was applied between the gate electrode and the Co layer. In our definition, the application of a positive (negative) V G resulted in an increase (decrease) in the electron density at the Co surface. Photographs of samples 1 and 2 are shown in Fig. 1b,c . 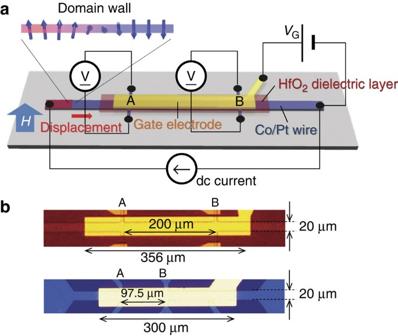Figure 1: Device structure and measurement configuration. (a) A schematic diagram of the device structure and the measurement configuration. The device consisted of a Co/Pt microwire, a HfO2dielectric layer, and a gate electrode on top. The Hall resistances at two Hall probes (a) and (b) were measured by applying a constant dc current to the perpendicularly magnetized Co/Pt (10 μA in sample 1 and 20 μA in sample 2). The Hall resistances were used to detect the magnetization direction in the vicinity of the probes when a perpendicular magnetic field and gate voltageVGwere applied.VGwas applied between the gate electrode and Co layer. (b) Photographs of sample 1 (upper) and sample 2 (lower). The samples had the same wire width (20 μm) but different distances between the Hall probes (a) and (b) (200 μm in sample 1 and 97.5 μm in sample 2). The Co layer was 0.4-nm thick in both samples and the Pt layer under it was 1.04-nm thick in sample 1 and 1.20-nm thick in sample 2. Figure 1: Device structure and measurement configuration. ( a ) A schematic diagram of the device structure and the measurement configuration. The device consisted of a Co/Pt microwire, a HfO 2 dielectric layer, and a gate electrode on top. The Hall resistances at two Hall probes ( a ) and ( b ) were measured by applying a constant dc current to the perpendicularly magnetized Co/Pt (10 μA in sample 1 and 20 μA in sample 2). The Hall resistances were used to detect the magnetization direction in the vicinity of the probes when a perpendicular magnetic field and gate voltage V G were applied. V G was applied between the gate electrode and Co layer. ( b ) Photographs of sample 1 (upper) and sample 2 (lower). The samples had the same wire width (20 μm) but different distances between the Hall probes ( a ) and ( b ) (200 μm in sample 1 and 97.5 μm in sample 2). The Co layer was 0.4-nm thick in both samples and the Pt layer under it was 1.04-nm thick in sample 1 and 1.20-nm thick in sample 2. Full size image The anomalous Hall effect was used to detect the local magnetization direction in the vicinity of the Hall probes [22] , [24] , [25] , [26] , [27] , [32] , [34] , [35] , [36] , [37] . The Hall resistance R Hall , which is proportional to the perpendicular component of the magnetization M , was measured under an external magnetic field H applied perpendicularly to the Co film (see Methods for the details of the transport measurement). 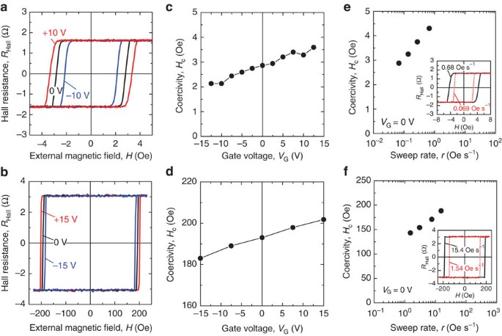Figure 2: Magnetic hysteresis loops and coercivity under various gate voltages. (a) and (b) The external magnetic fieldHdependences of Hall resistanceRHallat the Hall probe B for (a) sample 1 (290 K) and (b) sample 2 (295 K). The red, black, and blue curves respectively indicate the results obtained when applying gate voltagesVG+10, 0, and −10 V. The sweep rates ofHfor samples 1 and 2 were, respectively, 0.069 and 7.68 Oe s−1.RHallis proportional to the perpendicular component of magnetization because of the anomalous Hall effect. In both samples, clear modification of coercivity (Hc) is observed depending on the value of gate voltage (VG). (c) and (d) TheVGdependence of the coercivityHcfor (c) sample 1 at 290 K and (d) sample 2 at 295 K. The sweep rates ofHused to determineHcfor samples 1 and 2 were, respectively, 0.069 and 7.68 Oe s−1.Hcincreases withVG. (e) and (f) Magnetic-field sweep rate (r) dependence ofHcatVG=0 V for (e) sample 1 (290 K) and (f) sample 2 (300 K).Hcincreases withr. The insets shows the external magnetic fieldHdependence of Hall resistanceRHallat the Hall probe B atVG=0 V.rfor the measurements were indicated in the figure. Figure 2a,b show the R Hall vs H curves for samples 1 and 2 obtained applying three different V G . The electric field at | V G |=1 V corresponds to an electric field strength of ~0.2 MV cm −1 . In both samples, the coercivity ( H c ) clearly depended on the V G . The V G dependence of the values of the H c for samples 1 and 2 are shown in Fig. 2c,d . H c was increased (reduced) by applying positive (negative) V G . This result reproduces our previous results [37] . Figure 2: Magnetic hysteresis loops and coercivity under various gate voltages. ( a ) and ( b ) The external magnetic field H dependences of Hall resistance R Hall at the Hall probe B for ( a ) sample 1 (290 K) and ( b ) sample 2 (295 K). The red, black, and blue curves respectively indicate the results obtained when applying gate voltages V G +10, 0, and −10 V. The sweep rates of H for samples 1 and 2 were, respectively, 0.069 and 7.68 Oe s −1 . R Hall is proportional to the perpendicular component of magnetization because of the anomalous Hall effect. In both samples, clear modification of coercivity ( H c ) is observed depending on the value of gate voltage ( V G ). ( c ) and ( d ) The V G dependence of the coercivity H c for ( c ) sample 1 at 290 K and ( d ) sample 2 at 295 K. The sweep rates of H used to determine H c for samples 1 and 2 were, respectively, 0.069 and 7.68 Oe s −1 . H c increases with V G . ( e ) and ( f ) Magnetic-field sweep rate ( r ) dependence of H c at V G =0 V for ( e ) sample 1 (290 K) and ( f ) sample 2 (300 K). H c increases with r . The insets shows the external magnetic field H dependence of Hall resistance R Hall at the Hall probe B at V G =0 V. r for the measurements were indicated in the figure. Full size image To find out what determines the H c , we first checked the dependence of H c on the sweep rate of H ( r ) as shown for samples 1 and 2 in Fig. 2e,f . The results show that the H c significantly increases with r . This implies that H c is determined by a domain nucleation in the vicinity of the Hall probes, or the arrival of the DW at the Hall probe of a domain after the nucleation of a domain somewhere else in the wire. To find out which determines the H c , we conducted the following experiment. We prepared a single-domain state by applying a sufficiently large negative H , returned H to zero, and then measured the switching time of R Hall for the two Hall probes under a constant positive H . The result obtained in sample 2 at H =121 Oe is shown in Fig. 3a . The switching of the sign of the normalized R Hall from negative to positive was observed at both probes, and probe A switched before probe B. We repeated the same procedure under various H and found that probe A always switched before probe B regardless of the magnitude of H ( Supplementary Fig. S1 ). 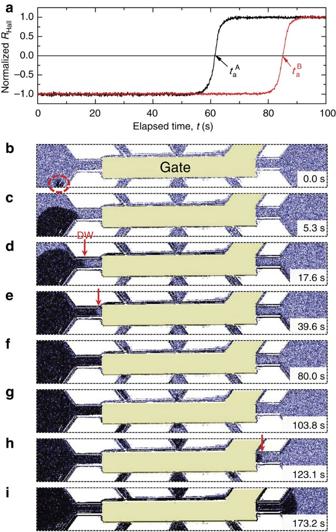Figure 3: Hall resistance switching due to arrival of domain wall and domain images obtained using a magneto-optical Kerr effect microscope. (a) Normalized Hall resistancesRHallat probes A (black line) and B (red line) as a function of the elapsed timetfor sample 2. The results shown here were obtained atVG=0 V and 295 K. Before measurement, a single-domain state was prepared by applying sufficiently large negativeH. The positive external magnetic fieldHof 121 Oe was applied att=0 s. Switching of the sign in the normalizedRHallfrom negative to positive indicates domain wall arrival at the probe. (b–i) Domain images obtained with a MOKE microscope after a single domain had been produced by applying a sufficiently large negativeH.H=+170 Oe was applied att=0 and was maintained for 5 s, nucleating a domain (indicated by the dashed red circle) and expanded it. Att=5 s,Hwas reduced to +120 Oe. After that the DW came into the wire. The series of images shows the DW creep motion from left to right along the wire. We thus inferred that the domain was nucleated somewhere outside the wire and then the DW entered the wire and travelled along it, arriving first at probe A and then at B with different arrival times, t a A and t a B Figure 3: Hall resistance switching due to arrival of domain wall and domain images obtained using a magneto-optical Kerr effect microscope. ( a ) Normalized Hall resistances R Hall at probes A (black line) and B (red line) as a function of the elapsed time t for sample 2. The results shown here were obtained at V G =0 V and 295 K. Before measurement, a single-domain state was prepared by applying sufficiently large negative H . The positive external magnetic field H of 121 Oe was applied at t =0 s. Switching of the sign in the normalized R Hall from negative to positive indicates domain wall arrival at the probe. ( b – i ) Domain images obtained with a MOKE microscope after a single domain had been produced by applying a sufficiently large negative H . H =+170 Oe was applied at t =0 and was maintained for 5 s, nucleating a domain (indicated by the dashed red circle) and expanded it. At t =5 s, H was reduced to +120 Oe. After that the DW came into the wire. The series of images shows the DW creep motion from left to right along the wire. Full size image MOKE measurement To confirm this inference, we obtained domain images by using the magneto-optical Kerr effect (MOKE). Before obtaining the images, we prepared a single-domain state by applying a sufficiently large negative field before returning it to zero. Then, a constant field of 170 Oe was applied (rise time 0.3 s) and the MOKE image was taken after the field reached its final value ( Fig. 3b ). In order to enhance the image contrast, the differential images before and after the application of a positive field are shown. The blue color in the image indicates that the magnetization in that region points toward the negative direction, and black indicates that the magnetization there points in the positive direction. An incidental nucleation of the domain at the position indicated by a dashed circle can be seen. Continued application of 170 Oe expanded the domain ( Fig. 3c ) until, at t =5 s, the magnetic field was reduced to H =120 Oe. The DW gradually came into the wire ( Fig. 3d ) and travelled along it ( Fig. 3e ). The DW motion under the gate ( Fig. 3f,g ) could not be seen, but the black region eventually appeared beyond the gate ( Fig. 3h ) and the domain continued to expand ( Fig. 3i ). Gate voltage dependence of the domain-wall velocity The MOKE images clearly show that the DW propagated from left to right, which is consistent with t a A < t a B . Therefore, the DW velocity v can be determined by using both the Hall measurement results ( v = d AB /( t a B − t a A ), where d AB is the distance between probes A and B (200 μm in sample 1 and 97.5 μm. in sample B)) and the MOKE images ( v = d G / Δt , where Δt is the travelling time of the DW under the gate and d G , the length of the gate (356 μm in sample 1 and 300 μm in sample 2)]. We determined v under various H and V G as described above ( Fig. 4a,b ). We confirmed that the v values determined both ways showed good agreement as shown in Fig. 4b . The V G dependence of the v determined from the Hall measurement is summarized for samples 1 and 2 in the insets of Fig. 4a,b , where the V G dependence of the v at different H is shown. In both samples, the v increased with V G was observed, and in sample 1, it increased by more than an order of magnitude. 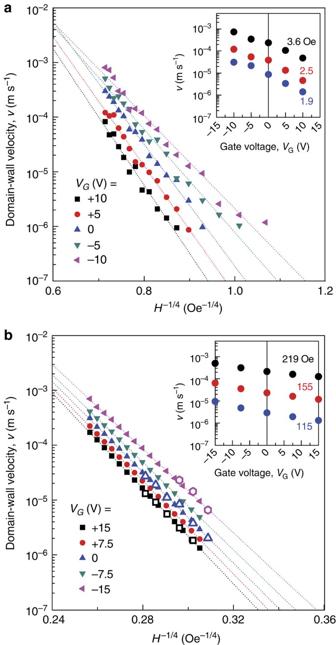Figure 4: Domain-wall velocity under the application of various gate voltages. The main panels show the DW velocityvas a function ofH−1/4under the application of five different gate voltagesVGfor (a) sample 1 (290 K) and (b) sample 2 (295 K). Filled symbols show thevdetermined by Hall measurement, and open symbols show thevdetermined from MOKE images. The inset shows theVGdependence ofvfor three differentHvalues (3.6 (black), 2.5 (red), and 1.9 Oe (blue) for sample 1, and 219 (black), 155 (red), and 115 Oe (blue) for sample 2). ChangingVGfrom −10 V to +10 V changedvby more than an order of magnitude. Figure 4: Domain-wall velocity under the application of various gate voltages. The main panels show the DW velocity v as a function of H −1/4 under the application of five different gate voltages V G for ( a ) sample 1 (290 K) and ( b ) sample 2 (295 K). Filled symbols show the v determined by Hall measurement, and open symbols show the v determined from MOKE images. The inset shows the V G dependence of v for three different H values (3.6 (black), 2.5 (red), and 1.9 Oe (blue) for sample 1, and 219 (black), 155 (red), and 115 Oe (blue) for sample 2). Changing V G from −10 V to +10 V changed v by more than an order of magnitude. Full size image The obtained v is in the range of ~10 −6 –10 −3 m s −1 , indicating that the DW motion is in the thermally activated creep regime. It is known that, in this regime, the DW velocity can be expressed as a function of H by using the following scaling function: where v 0 is a numerical prefactor, U c , the scaling energy constant, H crit , the critical field, μ , a universal dynamic exponent, k B , the Boltzmann constant, and T , the temperature. The U c is determined by the height of the disorder-induced DW pinning energy barrier, and the H crit is determined by the depinning field. It is known that μ is equal to 1/4 for a one-dimensional DW travelling in a weakly disordered two-dimensional medium like an ultrathin Co film [38] , [39] , [40] . To check the validity of equation (1) with μ =1/4, we plotted log v vs H 1/4 ( Fig. 4a,b ). The results indeed prove that in both samples linear behaviour is obtained at any values of V G , thus confirming the universality of μ (we also confirmed its universality at various temperatures ( Supplementary Fig. S2 )). The linear fittings to the results clearly have different slopes depending on V G , indicating that the effective critical field [39] , [43] , H eff =( U c / k B T ) 4 H crit , is a function of V G . The V G dependences of H eff for samples 1 and 2 (determined from the slopes of the linear fittings in Fig. 4a,b ) are shown in Fig. 5a,b . From these plots, one can see that H eff increases almost linearly with V G . This indicates that the energy barrier of the pinning potential randomly introduced in the wire is modulated electrically. 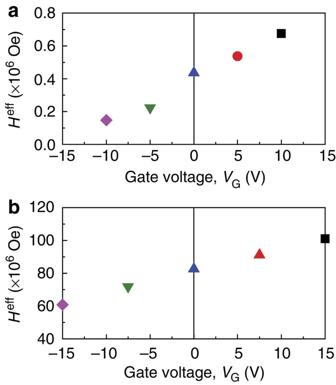Figure 5: Gate voltage dependence of effective critical field. Effective critical fieldHeffas a function ofVGfor (a) sample 1 (290 K) and (b) sample 2 (295 K).Heffincreases almost linearly withVG, indicating that the pinning energy barrier for the DW can be controlled. Figure 5: Gate voltage dependence of effective critical field. Effective critical field H eff as a function of V G for ( a ) sample 1 (290 K) and ( b ) sample 2 (295 K). H eff increases almost linearly with V G , indicating that the pinning energy barrier for the DW can be controlled. Full size image As the present measurements were carried out at temperatures slightly below the Curie temperature T C (at 0.91 T C for sample 1 (whose T C at V G =0 V was ~318 K), and at 0.76 T C for sample 2 (whose T C at V G =0 V was ~387 K); Supplementary Fig. S3 ), the modulation of T C by V G (ref. 37 ) is expected to lead to significant changes in the magnetic parameters that determine H eff especially the magnitudes of the saturation magnetization M s and the effective perpendicular anisotropy. One can assume that the DW velocity increases when the effective perpendicular anisotropy H u┴ eff is decreased by applying V G (refs 30 , 43 ). We checked that, at a constant V G , H u┴ eff and R Hall at zero field (and thus at remanent magnetization) decreased as temperature increased, and that U c ( H crit ) 1/4 (=( H eff ), 1/4 k B T ) also decreased with temperature, as shown in Fig. 6a (is the determination of the H u┴ eff is described in the Methods). This is consistent with the above assumption. At a constant temperature, however, the results were not straightforward: when a positive V G was applied, the U c ( H crit ) 1/4 increased but the H u┴ eff (including a diamagnetic field term) decreased ( Fig. 6b ). One possible explanation of the V G dependence of the H u┴ eff is that by applying positive V G increases the M s . That is, under the assumption that the perpendicular anisotropy constant K u is independent of V G , the H u┴ eff (= K u / M s −2 πM s ) might be reduced by an increase of M s , and thus the diamagnetic field (2 πM s ), when a positive V G is applied. One interesting result that supports the above speculation is shown in Fig. 7a,b : the average Hall resistance R Hall ave increased slightly with V G , and the average sheet resistance R sheet ave decreased with it. This may be an indication of the change in M s by V G , if we can assume that M s is proportional to R Hall ave /( R sheet ave ) γ , where γ is 1 or 2, although the direct measurement of M s under the gate is clearly needed to further understand the observed V G dependence of the DW velocity. Another fact we have confirmed is that U c ( H crit ) 1/4 could be scaled by 1− T / T C : the values obtained at different V G collapsed to a single curve when plotted against 1− T / T C ( Supplementary Fig. S4 ). 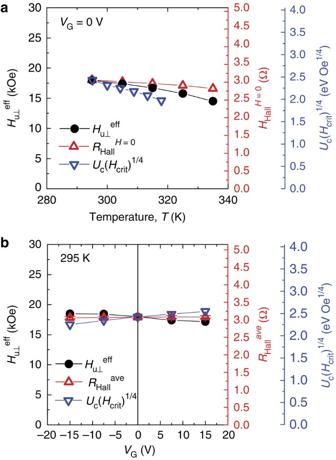Figure 6: Temperature and gate voltage dependences of effective perpendicular anisotropy andUc(Hcrit)1/4. (a) Temperature dependence of the effective perpendicular anisotropy fieldHu┴eff, the Hall resistance atH=0 Oe (RHallH=0), andUc(Hcrit)1/4atVG=0 V. (b)VGdependence of the effective perpendicular anisotropy fieldHueff, the averaged Hall resistanceRHallavedetermined fromRHallvalues in the saturated state of magnetization in the hysteresis loop, andUc(Hcrit)1/4. The results were obtained at 295 K using sample 2. Figure 6: Temperature and gate voltage dependences of effective perpendicular anisotropy and U c ( H crit ) 1/4 . ( a ) Temperature dependence of the effective perpendicular anisotropy field H u┴ eff , the Hall resistance at H =0 Oe ( R Hall H =0 ), and U c ( H crit ) 1/4 at V G =0 V. ( b ) V G dependence of the effective perpendicular anisotropy field H u eff , the averaged Hall resistance R Hall ave determined from R Hall values in the saturated state of magnetization in the hysteresis loop, and U c ( H crit ) 1/4 . The results were obtained at 295 K using sample 2. 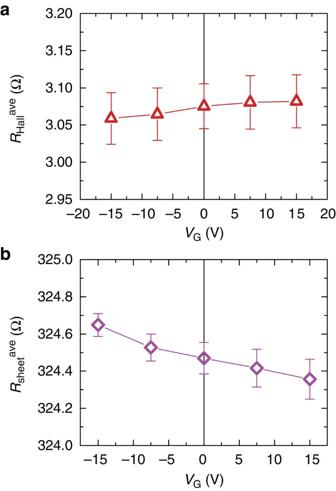Figure 7: Gate voltage dependence of the Hall resistance and the sheet resistance. (a)VGdependence of theRHallavedetermined fromRHallvalues in the saturated state of magnetization in the hysteresis loop. (b)VGdependence of theRsheetavedetermined from theHdependence ofRsheetvalues. The error bars were s.d. of 100 data points. The results were obtained in sample 2 at 295 K. Full size image Figure 7: Gate voltage dependence of the Hall resistance and the sheet resistance. ( a ) V G dependence of the R Hall ave determined from R Hall values in the saturated state of magnetization in the hysteresis loop. ( b ) V G dependence of the R sheet ave determined from the H dependence of R sheet values. The error bars were s.d. of 100 data points. The results were obtained in sample 2 at 295 K. Full size image In summary, we have demonstrated that the DW velocity can be changed by more than an order of magnitude through the application of electric fields. The effective critical field was revealed to be a function of V G , meaning that the energy barrier for thermally activated DW motion is electrically controllable. We think that the concept presented here will be useful in reducing the energy consumption of magnetic recording media and logic devices and that investigating the effects of electric fields on the DW displacement induced by electric currents will provide additional knowledge useful for understanding the physics underlying the universal behaviour of the DW creep [18] as well as for developing practical devices. Film deposition The films from which the present wire devices were made were deposited by dc and rf sputtering. A 0.4-nm thick Co layer with a 2.0-nm thick MgO cap layer was deposited on a semi-insulating GaAs (001) substrate. Under the Co layer were a Pt layer (1.04 nm thick in sample 1 and 1.20 nm thick in sample 2) and, below that, a Ta layer with 3.0 nm thick. Layer thickness was determined from the deposition rate of each material. Device fabrication The field-effect devices we used here were fabricated as follows. After photolithography and Ar ion milling were used to make a 20-μm wide Co wire with two Hall probes (A and B), atomic layer deposition was used to cover the wire with a 50-nm thick HfO 2 gate insulator (the deposition was carried out in the atomic layer deposition chamber, Savannah K-100, Cambridge NanoTech.). Finally, a lift-off process was used to form the Au (47 nm)/Cr (3 nm) gate electrode. Hall resistance measurement A Helmholtz coil was used to apply an external magnetic field H normal to the film surface, and a dc current was applied to detect the Hall resistance ( R Hall ). The magnitude of dc current was 20 μA for sample 1 and 10 μA for sample 2. The density of the current flowing in the Co layer is 1.6×10 8 A m −2 in sample 1 and 0.8×10 8 A m −2 in sample 2. We confirmed that the creep velocity was independent of the direction of the detection current ( Supplementary Fig. S5 ). Determination of the effective perpendicular anisotropy The effective perpendicular anisotropy H u┴ eff was determined from the saturation field of the magnetization by applying in-plane magnetic fields H in−plane , hard-axis fields. 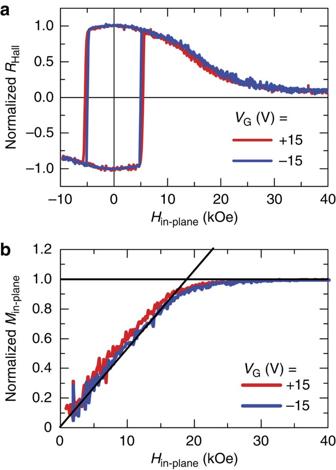Figure 8: Determination of the effective perpendicular anisotropy field. (a) In-plane magnetic fieldHin−planedependence of the normalized Hall resistance whenVG=+15 and −15 V were applied in sample 2 at 295 K. (b)Hin−planedependence of the normalized in-plane component of the magnetizationMin−planedetermined from the normalized Hall resistance forVG=−15 and +15 V. The intersection of the two black lines gives the effective perpendicular anisotropy fieldHu┴eff. Figure 8a shows the normalized R Hall ( R Hall norm ) as a function of H in−plane . The R Hall norm at H in−plane =0 Oe (positive one) decreases with increasing H in−plane , indicating that the magnetization tilted from the perpendicular to the in-plane direction. The normalized in-plane component of the magnetization ( M in−plane ) can be determined from R Hall norm by using the following relation: M in−plane / M s =sin{cos −1 ( R Hall norm )}, and the result is shown in Fig. 8b . H u┴ eff was determined from the intersection of the two black lines there. Figure 8: Determination of the effective perpendicular anisotropy field. ( a ) In-plane magnetic field H in−plane dependence of the normalized Hall resistance when V G =+15 and −15 V were applied in sample 2 at 295 K. ( b ) H in−plane dependence of the normalized in-plane component of the magnetization M in−plane determined from the normalized Hall resistance for V G =−15 and +15 V. The intersection of the two black lines gives the effective perpendicular anisotropy field H u┴ eff . Full size image How to cite this article: Chiba, D. et al . Electric-field control of magnetic domain-wall velocity in ultrathin cobalt with perpendicular magnetization. Nat. Commun. 3:888 doi: 10.1038/ncomms1888 (2012).